In situnanoindentation study on plasticity and work hardening in aluminium with incoherent twin boundaries Nanotwinned metals have been the focus of intense research recently, as twin boundaries may greatly enhance mechanical strength, while maintaining good ductility, electrical conductivity and thermal stability. Most prior studies have focused on low stacking-fault energy nanotwinned metals with coherent twin boundaries. In contrast, the plasticity of twinned high stacking-fault energy metals, such as aluminium with incoherent twin boundaries, has not been investigated. Here we report high work hardening capacity and plasticity in highly twinned aluminium containing abundant Σ3{112} incoherent twin boundaries based on in situ nanoindentation studies in a transmission electron microscope and corresponding molecular dynamics simulations. The simulations also reveal drastic differences in deformation mechanisms between nanotwinned copper and twinned aluminium ascribed to stacking-fault energy controlled dislocation-incoherent twin boundary interactions. This study provides new insight into incoherent twin boundary-dominated plasticity in high stacking-fault energy twinned metals. Nanotwinned (nt) metals stirred significant interest lately because Σ3{111} coherent twin boundaries (CTBs) contribute to high strength and ductility [1] , [2] , [3] , [4] , [5] , [6] , [7] , enhanced electrical conductivity [8] and superior thermal stability [9] . Plastic deformation mechanisms have been intensively studied in nt metals with face-centered cubic structure. The majority of prior studies focused on metals with low stacking-fault energy (SFE) (Cu, Ag) and/or a low ratio of unstable twinning ( γ ut ) to unstable stacking energy ( γ us ), because twins readily form in such metals during growth or deformation [10] , [11] , [12] , [13] . Although the density of incoherent twin boundaries (ITBs) is typically lower than that of CTBs, both CTBs and ITBs have been found to play crucial roles in plastic deformation in nt metallic materials with low SFE; CTBs act as barriers for slip, but ITBs can easily migrate in association with detwinning [14] , [15] . Furthermore, the deformation mechanisms of nt metals with extremely fine nanotwins are dominated by Shockley partial dislocations [4] , which are mostly nucleated from ITBs. Hence, it is critical to understand the role of ITBs in the deformation behaviour of nt metals. Atomistic simulations also predicted the dependence of deformation mechanisms on SFE in high SFE nt metals [16] . Validation of such predictions has not been accomplished, as fabrication of high-density growth twins in metals with high SFE and high γ ut / γ us ratio has proven to be difficult. For example, in Al, deformation twins only form sporadically under extreme conditions, such as near crack tips (high stress concentration), during ball milling at cryogenic temperature or in deformed nanocrystalline grains [17] , [18] , [19] , [20] . While mechanical behaviour of conventional polycrystalline Al has been studied, including pop-in effects [21] , stress-induced grain boundary migration [22] , the onset of plasticity before the first increase in repulsive force [23] , reverse dislocation motion on unloading [24] and strain rate-dependent plasticity [25] , successful fabrication of high-density growth twins in Al was only recently accomplished [26] , [27] ; thus, the deformation behaviour of highly twinned Al remains a mystery. In the present study, we use an in situ nanoindentation technique (inside a transmission electron microscope) and molecular dynamics (MD) simulations to show that ITBs enable significant work hardening and plasticity in highly twinned Al. ITBs are formidable barriers against the pile-up of dislocations, and thus may induce significant work hardening and high strength in twinned Al. The formation of steps on ITBs facilitates the transmission of dislocations, and these ITB steps can migrate at higher stresses to sustain plasticity. In comparison with extensive prior studies on CTB-dictated plasticity in low SFE metals, this study provides a fresh perspective towards understanding of ITB-dominated strengthening and plasticity in high SFE twinned metals. Dislocation nucleation and absorption by ITBs Epitaxial {111} nt Al films fabricated by magnetron sputtering contained abundant ITBs and occasional CTBs (See Methods and Supplementary Fig. 1a,b ). High-resolution transmission electron microscopy (TEM) micrographs ( Supplementary Fig. 1c,d ) reveal the atomic arrangement of a straight ITB. The average domain size is ~200 nm. ITBs become dominant defects in as-deposited highly twinned Al films, hence an opportunity to fully characterize their role in deformation physics of high SFE metals emerges. The cross-section TEM micrograph in Fig. 1a shows a straight ITB separating two domains, and the inset selected area diffraction patterns reveal the twinned orientation between these domains. Multiple indentation cycles were performed at this location to investigate deformation mechanisms. During the first indentation cycle ( Supplementary Movie 1 ), a prominent non-linear deformation regime was identified at ~75 MPa ( Fig. 1b ), followed by substantial work hardening. Even slight contact from the indenter tip removed small pre-existing dislocation loops ( Fig. 1c ). As indentation progressed, two threading dislocations first retracted from the surface, then formed a tangle ( Fig. 1d ), which continued to evolve under stress ( Fig. 1e,f ). At 45.9 s, dislocation bursts accompanied by prominent load drops occurred ( Fig. 1g ). After indentation ( Fig. 1h ), the affected volume beneath the indenter was cleared of many small dislocations, with the remaining large sessile defects. 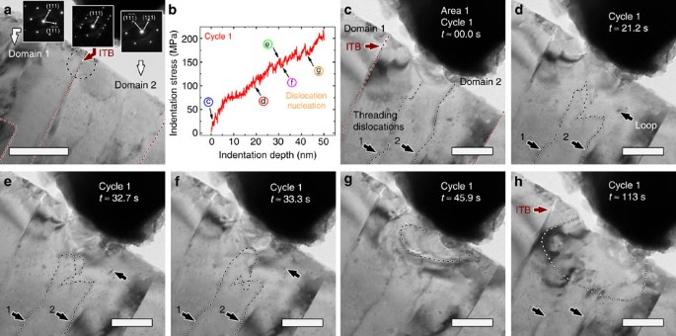Figure 1: Dislocation nucleation-dominated work hardening in nt Al. (a) Cross-section bright-field TEM micrograph of nt Al (near Alzone axis) showing an overview of the area of interest before indentation. Scale bar, 200 nm. (b) Indentation stress as a function of indentation depth for indentation cycle 1. The onset of plastic yielding occurred at ~75 MPa. (c) Before indentation, two grown-in threading dislocations extended to the film surface. Scale bar for this and subsequent panels is 100 nm. (d) At 21.2 s, threading dislocations 1 and 2 retracted rapidly and formed a tangle. (e,f) By 32.7 s, dislocations 1 and 2 continued to evolve, while small loops migrated (arrows). (g) Whent≈45.9 s, a dislocation burst occurred. (h) By 113 s, after indentation, many small defects were removed from the activated volume, and only larger sessile loops remained (SeeSupplementary Movie 1). Figure 1: Dislocation nucleation-dominated work hardening in nt Al. ( a ) Cross-section bright-field TEM micrograph of nt Al (near Al zone axis) showing an overview of the area of interest before indentation. Scale bar, 200 nm. ( b ) Indentation stress as a function of indentation depth for indentation cycle 1. The onset of plastic yielding occurred at ~75 MPa. ( c ) Before indentation, two grown-in threading dislocations extended to the film surface. Scale bar for this and subsequent panels is 100 nm. ( d ) At 21.2 s, threading dislocations 1 and 2 retracted rapidly and formed a tangle. ( e , f ) By 32.7 s, dislocations 1 and 2 continued to evolve, while small loops migrated (arrows). ( g ) When t ≈45.9 s, a dislocation burst occurred. ( h ) By 113 s, after indentation, many small defects were removed from the activated volume, and only larger sessile loops remained (See Supplementary Movie 1 ). Full size image The stress–displacement plot from the second indentation cycle in Fig. 2a shows plastic yielding at ~180 MPa followed by a series of rapid load drops. The labelled arrows correspond to the succeeding micrographs in Fig. 2b–g (also see Supplementary Movie 2 ). At the beginning of cycle 2, only a few sessile loops (black arrows) remained ( Fig. 2b ). At 19.9 s, plastic yielding occurred ( Fig. 2c ); a dislocation (dotted line) nucleated beneath the indenter accompanied by strain contours (open arrows), and the indentation curve deviated from linearity. Preceding the stress drop ( Fig. 2d ), several sessile loops (black arrows) were present beneath the indenter. A sudden dislocation avalanche at 42.6 s ( Fig. 2e ) resulted in a prominent strain burst outlined by a group of large circular dislocation loops accompanied by a substantial load drop. Small sessile dislocation loops pinned the right side of the large loops, while the straight ITB pinned their left. These dislocation loops propagated outward ( Fig. 2f ), and were partially absorbed by the ITB; however, no dislocations penetrated the ITB during this entire cycle. 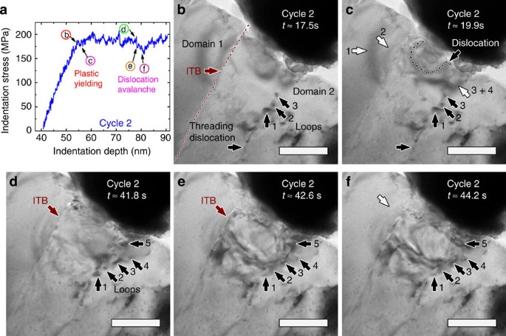Figure 2: The nucleation and avalanche of dislocations confined by the ITB. (a) Indentation stress–displacement curve from indentation cycle 2, with arrows indicating the location of events recorded in the following micrographs. (b)t≈17.5 s: elastic deformation regime. The ITB, threading dislocation tangle and dislocation loops (labelled by black arrows) fromFig. 1were still present. Scale bar in this and subsequent panels is 100 nm. (c)t≈19.9 s: yielding. Dislocations (indicated by a dotted line) emerged and propagated downward from the indenter. (d)t≈41.8 s: just before a distinct stress drop, dislocations were active beneath the indenter and several sessile loops had been generated (labelled by black arrows). (e)t≈42.6 s: in less than one frame, an oval-shaped avalanche of large dislocations (~130 nm in diameter) appeared, accompanied by a substantial load drop. Loops were pinned by sessile dislocation loops (arrows 1–5) on the right and blocked by the ITB on the left. (f)t≈44.2 s: the dislocations propagating rightward interacted with small sessile loops. However, those dislocations propagating leftward were absorbed by the ITB. No dislocations crossed the ITB during this indentation cycle. (SeeSupplementary Movie 2). Figure 2: The nucleation and avalanche of dislocations confined by the ITB. ( a ) Indentation stress–displacement curve from indentation cycle 2, with arrows indicating the location of events recorded in the following micrographs. ( b ) t ≈17.5 s: elastic deformation regime. The ITB, threading dislocation tangle and dislocation loops (labelled by black arrows) from Fig. 1 were still present. Scale bar in this and subsequent panels is 100 nm. ( c ) t ≈19.9 s: yielding. Dislocations (indicated by a dotted line) emerged and propagated downward from the indenter. ( d ) t ≈41.8 s: just before a distinct stress drop, dislocations were active beneath the indenter and several sessile loops had been generated (labelled by black arrows). ( e ) t ≈42.6 s: in less than one frame, an oval-shaped avalanche of large dislocations (~130 nm in diameter) appeared, accompanied by a substantial load drop. Loops were pinned by sessile dislocation loops (arrows 1–5) on the right and blocked by the ITB on the left. ( f ) t ≈44.2 s: the dislocations propagating rightward interacted with small sessile loops. However, those dislocations propagating leftward were absorbed by the ITB. No dislocations crossed the ITB during this indentation cycle. (See Supplementary Movie 2 ). Full size image Significant work hardening in highly twinned Al During the third indentation cycle, the indentation stress–displacement curve in Fig. 3a shows apparent work hardening behaviour. Multiple arrows placed on each side of the curve and the adjacent letters correspond to the following TEM micrographs. During elastic deformation up to 10 s ( Fig. 3b ), several pre-existing dislocations (mostly residual dislocations from prior indentation cycles) started to migrate toward the ITB. Domain 2 underneath the indenter maintained its low dislocation density. By 29 s ( Fig. 3c ), preceding the onset of stress drop shown in Fig. 3a , these pre-existing dislocations formed a network and piled up at the ITB, denoted by a red dotted line. At 33 s as shown in Fig. 3d , instantaneous nucleation of numerous dislocations occurred corresponding to the distinctive load drop at point d in Fig. 3a . By 37 s ( Fig. 3e ), the new dislocations propagated left toward the ITB where they were obstructed. By 40 s, the continuous pile-up of dislocations appeared to distort a small portion of the ITB (forming step 1) as indicated by a red dotted line in Fig. 3f . During further indentation at increasing stress levels ( Fig. 3g–i ), more dislocations piled up against the ITB, and consequently the ITB became further distorted as shown by the additional red dotted line (delineating step 2 and 3 on the ITB). Note that during the work hardening process, the deformation-induced dislocation activities (nucleation and pile ups) were entirely self-contained in domain 2, and no dislocations were able to breach the ITB obstacle. (See Supplementary Movie 3 for more detail). 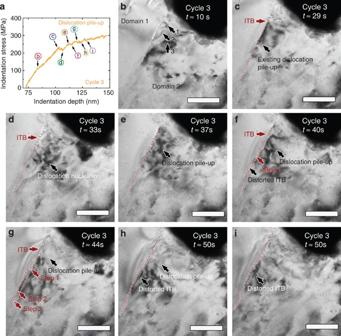Figure 3: Dislocation pile-ups against ITBs and work hardening. (a) The indentation stress–displacement curve during indentation cycle 3 shows work hardening behaviour. Multiple arrows placed on each side of the curve and the adjacent letters correspond to the following TEM micrographs. (b) During elastic deformation up to 10 s, several pre-existing dislocations started to migrate toward the ITB. The domain 2 underneath the indenter remained its low dislocation density. Scale bar here and in subsequent panels is 100 nm. (c) By 29 s, right before the onset of load drop (shown ine), the pre-existing dislocations formed a network and piled up at the ITB, the position of which was outlined by a red dotted line. (d) At 33 s, instantaneous nucleation of numerous dislocations occurred, and the nucleation event was accompanied by a distinctive load drop. (e) At 37 s, these new dislocations propagated left toward the ITB whereat they were blocked. (f) By 40 s, the continuous pile-up of dislocations appeared to distort a small portion of the ITB as indicated by a red dotted line labelled as step 1. (g–i) During further indentation at increasing stress levels, more dislocations piled up at the ITB. The ITB became increasingly distorted as shown by the additional red dotted line and steps 2 and 3 on the ITB are visible. Note that during this work hardening process, the dislocation activities remained in domain 2 exclusively as all dislocation pile-ups were stopped by the ITB (SeeSupplementary Movie 3). Figure 3: Dislocation pile-ups against ITBs and work hardening. ( a ) The indentation stress–displacement curve during indentation cycle 3 shows work hardening behaviour. Multiple arrows placed on each side of the curve and the adjacent letters correspond to the following TEM micrographs. ( b ) During elastic deformation up to 10 s, several pre-existing dislocations started to migrate toward the ITB. The domain 2 underneath the indenter remained its low dislocation density. Scale bar here and in subsequent panels is 100 nm. ( c ) By 29 s, right before the onset of load drop (shown in e ), the pre-existing dislocations formed a network and piled up at the ITB, the position of which was outlined by a red dotted line. ( d ) At 33 s, instantaneous nucleation of numerous dislocations occurred, and the nucleation event was accompanied by a distinctive load drop. ( e ) At 37 s, these new dislocations propagated left toward the ITB whereat they were blocked. ( f ) By 40 s, the continuous pile-up of dislocations appeared to distort a small portion of the ITB as indicated by a red dotted line labelled as step 1. ( g – i ) During further indentation at increasing stress levels, more dislocations piled up at the ITB. The ITB became increasingly distorted as shown by the additional red dotted line and steps 2 and 3 on the ITB are visible. Note that during this work hardening process, the dislocation activities remained in domain 2 exclusively as all dislocation pile-ups were stopped by the ITB (See Supplementary Movie 3 ). Full size image Dislocation transmission across ITBs Sequential TEM micrographs in Fig. 4a–d (also see Supplementary Movie 4 ) from the fourth indentation cycle illustrate the first dislocation transmission event across the ITB. The yield stress had increased to ~300 MPa ( Fig. 4a ) due to strain hardening from previous loading cycles. Just before transmission ( Fig. 4b ), numerous dislocations had piled up against the ITB, forming a dense dislocation network. Note that the initially straight ITB had formed a double kink ( Fig. 4b ) after repetitive interactions with dislocations during previous cycles. During subsequent loading, a dislocation emerged from the step 1 into domain 1 ( Fig. 4c ), and then quickly propagated leftward, depositing a loop by 56.6 s ( Fig. 4d ). The schematic in Fig. 4e shows the orientations of the adjacent domains, ITB, and slip systems. Compiled indentation stress–displacement curves for four consecutive indentation cycles at the same location in Fig. 4f show the cumulative work hardening behaviour in nt Al (See Supplementary Fig. 2 for the original load-displacement plots). 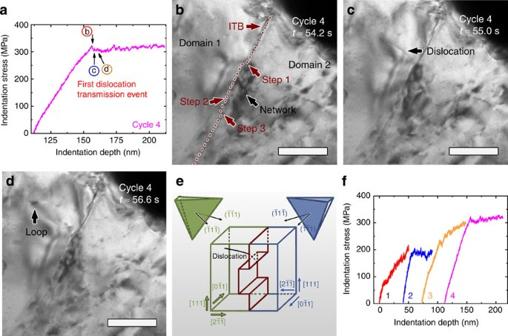Figure 4: Dislocation transmission event across the distorted ITB. (a) Corresponding stress–displacement curve with arrows indicating the following TEM micrographs. (b) At 54.2 s, the ITB had developed a double kink (dotted line). At the onset of plastic deformation (~300 MPa), numerous dislocations had piled up against the ITB. Scale bar in panelsb–dis 100 nm. (c) By 55.0 s, in one frame, a dislocation emerged from step 1 was emitted into domain 1. (d) At 56.6 s, the dislocation then propagated leftward within domain 1, leaving behind a dislocation loop. (e) Schematic showing orientations of the twin and matrix separated by an ITB. (f) Compiled curves for several cycles of successive indentations at the same location showing nominal indentation stress as a function of indentation depth. Note the classical work hardening behavior and numerous stress drops in the post-yielding regions of each curve. (SeeSupplementary Movie 4). Figure 4: Dislocation transmission event across the distorted ITB. ( a ) Corresponding stress–displacement curve with arrows indicating the following TEM micrographs. ( b ) At 54.2 s, the ITB had developed a double kink (dotted line). At the onset of plastic deformation (~300 MPa), numerous dislocations had piled up against the ITB. Scale bar in panels b – d is 100 nm. ( c ) By 55.0 s, in one frame, a dislocation emerged from step 1 was emitted into domain 1. ( d ) At 56.6 s, the dislocation then propagated leftward within domain 1, leaving behind a dislocation loop. ( e ) Schematic showing orientations of the twin and matrix separated by an ITB. ( f ) Compiled curves for several cycles of successive indentations at the same location showing nominal indentation stress as a function of indentation depth. Note the classical work hardening behavior and numerous stress drops in the post-yielding regions of each curve. (See Supplementary Movie 4 ). Full size image Migration of ITBs At even greater applied stress levels, substantial ITB migration occurred. 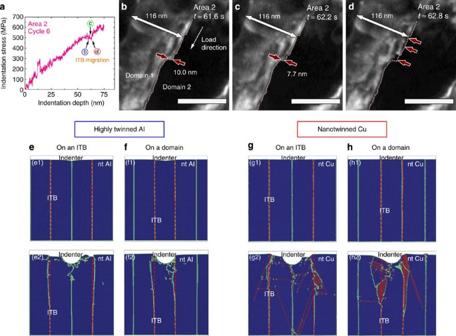Figure 5: ITB Migration and sliding in Al compared to ITB dissociation in Cu. (a–d) Substantial ITB migration during indentation in a second area. (a) Stress–displacement curve after five prior indentation cycles, with arrows indicating the points of interest in the succeeding TEM micrographs. (b) Whent≈61.6 s, a dark-field TEM micrograph taken just before ITB migration shows an ITB/CTB junction forming a corner and step approximately 10 nm wide. Scale bar in panelsb–dis 100 nm. (c) At 62.2 s, in less than one frame, the indicated ITB segment moved leftward, reducing the step to a width of ~7.7 nm, corresponding to a plateau of the stress–displacement curve inFig. 5a. (d) By 62.8 s, the ITB segment moved leftward again, removing the remaining step that is 7.7 nm wide. The dotted red line indicates the initial ITB position. Arrows indicate the location of the large migration event, as well as two smaller events above. (e–h) MD simulations of nanoindentation of nt Al and nt Cu with abundant ITBs at different locations using a fully elastic spherical indenter tip. Atoms are coloured according to Common-Neighbor Analysis (red-stacking fault; blue-normal face-centred cubic; green-defected face-centred cubic structure). (e,f) Comparison of the initial and deformed microstructures of nt Al when indenter was placed on an ITB (e1,e2), and inside a domain (f1,f2). Simulations show ITB migration and vertical sliding via interface dislocations, interaction of lattice dislocations emitted under indenter tip with ITBs and ITB migration. In particular, two kinks were observed on the deformed ITBs (e2,f2), and dislocations were confined by the ITBs, that is, plasticity is highly localized inside the domain (SeeSupplementary Fig. 5). The position of the indenter relative to the ITBs leads to insignificant change on the deformation physics of nt Al. (g,h) Comparison of the initial and deformed nt Cu when indentation was performed right on top of an ITB (g1,g2) or inside a domain (h1,h2). MD simulations show that (i) ITB dissociates rapidly into 9R phase, (ii) ITB migrates substantially and horizontally, but does not slide vertically and (iii) dislocations transmitted across ITBs frequently.Supplementary Movies 5 and 6are provided corresponding toFig. 5e(for nt Al) andFig. 5g(for nt Cu) respectively. Figure 5a–d illustrates a second set of indentations (in dark-field TEM mode) performed at a location different from those in Figs 1 , 2 , 3 , 4 . Before this indentation, five consecutive indentation cycles were performed in the same area, such that work hardening allowed the sample to reach much higher yield stress, as shown in Fig. 5a . A dark-field TEM micrograph captured at 61.6 s in Fig. 5b shows the area of interest just before the ITB migration event at ~500 MPa. The dotted line delineates the initial domain boundary position. A 10-nm wide step was visible; from here, a small segment of the ITB migrated leftward ~2.3 nm by 62.2 s ( Fig. 5c ), then another 7.7 nm by 62.8 s ( Fig. 5d ), accompanied by a prominent load drop ( Fig. 5a ). Figure 5: ITB Migration and sliding in Al compared to ITB dissociation in Cu. ( a – d ) Substantial ITB migration during indentation in a second area. ( a ) Stress–displacement curve after five prior indentation cycles, with arrows indicating the points of interest in the succeeding TEM micrographs. ( b ) When t ≈61.6 s, a dark-field TEM micrograph taken just before ITB migration shows an ITB/CTB junction forming a corner and step approximately 10 nm wide. Scale bar in panels b – d is 100 nm. ( c ) At 62.2 s, in less than one frame, the indicated ITB segment moved leftward, reducing the step to a width of ~7.7 nm, corresponding to a plateau of the stress–displacement curve in Fig. 5a . ( d ) By 62.8 s, the ITB segment moved leftward again, removing the remaining step that is 7.7 nm wide. The dotted red line indicates the initial ITB position. Arrows indicate the location of the large migration event, as well as two smaller events above. ( e – h ) MD simulations of nanoindentation of nt Al and nt Cu with abundant ITBs at different locations using a fully elastic spherical indenter tip. Atoms are coloured according to Common-Neighbor Analysis (red-stacking fault; blue-normal face-centred cubic; green-defected face-centred cubic structure). ( e , f ) Comparison of the initial and deformed microstructures of nt Al when indenter was placed on an ITB (e1,e2), and inside a domain (f1,f2). Simulations show ITB migration and vertical sliding via interface dislocations, interaction of lattice dislocations emitted under indenter tip with ITBs and ITB migration. In particular, two kinks were observed on the deformed ITBs (e2,f2), and dislocations were confined by the ITBs, that is, plasticity is highly localized inside the domain (See Supplementary Fig. 5 ). The position of the indenter relative to the ITBs leads to insignificant change on the deformation physics of nt Al. ( g , h ) Comparison of the initial and deformed nt Cu when indentation was performed right on top of an ITB (g1,g2) or inside a domain (h1,h2). MD simulations show that (i) ITB dissociates rapidly into 9R phase, (ii) ITB migrates substantially and horizontally, but does not slide vertically and (iii) dislocations transmitted across ITBs frequently. Supplementary Movies 5 and 6 are provided corresponding to Fig. 5e (for nt Al) and Fig. 5g (for nt Cu) respectively. Full size image Next, we will discuss several key events associated with ITB-dominated plasticity in nt Al, including dislocation nucleation, strain hardening, ITB-dislocation interactions including pile ups and transmission and ITB migration. During in situ nanoindentation of highly twinned Al, we observed serrated stress drops, the magnitude of which substantially exceeded the noise level. These features are observed via the displacement-controlled indentation (as in this study), whereas strain bursts appear in force-controlled indentation [28] . Strain bursts have been frequently observed during micropillar compression tests of various metallic materials and have long been recognized as a consequence of dislocation nucleation events [29] , [30] . In the current nanoindentation studies of highly twinned Al, each strain burst was typically correlated to the nucleation of dislocations. The stress drop associated with most strain burst events was generally low, 10–20 MPa, as only individual dislocations were nucleated. However, during dislocation avalanches, sizable semicircular dislocation loops nucleated (for example, Figs 1g and 2e ), accompanied by substantial stress drops ( Figs 1b and 2a ), approaching 50 MPa in some cases. Interestingly, MD simulations [14] , [31] , [32] also predicted serrated stress-strain curve in nt Al, drastically different from that in low SFE nt Cu or Ag. Discrete dislocation dynamics simulations predicted that dislocation avalanches are a universal phenomenon during deformation of single-crystal Al, and grain boundaries in polycrystalline Al would reduce avalanche frequency [33] . Micropillar compression tests on Al yield controversial results [34] , [35] presumably related to the orientation of grain boundaries. The initial dislocation density in nt Al was low, and subsequent deformation at greater stress triggered frequent nucleation events, suggesting dislocation nucleation-dominated strain hardening in nt Al during early stages of deformation. Huang, et al ., observed annealing-induced hardening in commercial purity Al, and attributed such hardening to the depletion of mobile dislocation sources by annealing [36] . Meanwhile single-crystal micropillars with smaller diameter are typically stronger than those with larger diameters due presumably to dislocation starvation [29] , [37] . Interestingly, during indentation cycle 2, ITB began to absorb dislocations, that is, the ITB acted as a defect sink. Correspondingly, the stress–displacement curve flattened. The direct observation of dislocation absorption by ITBs validates a prior hypothesis by Kunz et al . [34] that ITBs might be defect sinks formulated from ex situ compression studies of Al micropillars. However, both Kunz et al . [34] and Ng and Ngan [35] were puzzled by the lack of dislocation pile ups along grain boundaries in deformed Al micropillars. This may be because their TEM samples were taken from excessively deformed micropillars. Our in situ movie shows that the ITB eventually lost its ability to absorb dislocations, followed by pile-up of dislocations against the ITB. Consequently, work hardening resumed in indentation cycles 3 and 4. To investigate the details of ITB-dislocation interactions, we performed large-scale MD simulations of nanoindentation near ITBs in twinned Al, where the fully elastic spherical indenter was positioned at the middle of a column and on top of an ITB, respectively ( Fig. 5e,f ). Atoms are coloured by using common-neighbor analysis. Our studies show that the position of the indenter relative to ITBs has insignificant impact on deformation physics of highly twinned Al. Thus, we summarize major findings by using simulation results from Fig. 5e1 (see Supplementary Movie 5 ). (1) During indentation, it is clear that lattice dislocations in nt Al nucleated in the region under the indenter, and migrated toward the ITBs. (2) Lattice dislocations met ITBs and then dissociated into interface disconnections [14] . The interface disconnection has a Burgers vector of and a step height of one atomic plane (see Supplementary Figs 3 and 4 for detail). This process resulted in the reduction of stress concentration compared with a non-dissociated lattice dislocation which delay slip transmission across an ITB. (3) The coupled shear migration of ITBs in the vertical {111} direction was observed, in addition to formation of horizontal steps at the ITB-dislocation interaction site ( Fig. 5f ). Coupled shear migration of ITBs also occurred in the top portion of the two ITBs where the interface disconnections protruded from the surface ( Fig. 5f ). Note that the formation of two kinks on a deformed ITB ( Fig. 5e2 ) is consistent qualitatively with in situ nanoindentation studies ( Fig. 3f–i ). Furthermore, simulations show that the dislocations were confined by the ITBs, in good agreement with substantial work hardening in nt Al discovered experimentally. In a second simulation, we used a twinned bicrystal model for Al to examine interface disconnection formation by single dislocations in detail (See Supplementary Figs 3 and 4 ). Three 60° mixed dislocations move towards an ITB under shear stress of 200 MPa at 10 K ( Fig. 4a ). Nucleation of the interface disconnection results from dissociation of the 60° mixed dislocation at the ITB ( Supplementary Fig. 4b–f ), which is described as . The residual component remains on the ITB plane, and appears as a step ( Supplementary Fig. 4e,f ). Hence, lattice dislocations were not able to penetrate ITBs due to the inherently high resistance of ITBs to the dissociation of dislocations. These MD simulations thus lend more support for the observed work hardening in twinned Al induced by ITBs. For comparison, we also performed MD simulations for similarly structured low SFE nt Cu where the fully elastic spherical indenter was located either on top of an ITB ( Fig. 5g1 , see Supplementary Movie 6 for detail) or on a domain ( Fig. 5h1 ). Again the mechanisms of deformation are insensitive to the location of indenter tip. MD simulations show that before absorption of the lattice dislocations, ITBs migrated and dissociated into two tilt walls bounding a volume of 9R phase [38] due to applied shear stress. The dissociation of ITBs is associated with crystal rotation of ~13° (ref. 14 ). The successive extension of 9R regions can accommodate plastic deformation in nt Cu. Meanwhile, dislocations transmit across ITBs easily at low stresses [39] . Thus, the ITB barrier resistance for lattice dislocations in nt Cu may not be as significant as those in nt Al. Continued dislocation-ITB interactions in twinned Al led to accumulation of residual dislocations, which appeared as steps along the initially straight ITB ( Fig. 4b ), consistent with MD simulations. These steps eventually grew pronounced enough to provide sites for dislocation transmission across the ITB or the nucleation of dislocations in the adjacent grain (see Supplementary Movie 5 for detail), that is, global plastic yielding (across multiple domains) occurred. The stress at which such a transmission event occurred was ~300 MPa, comparable to hardness of nt Al films measured by ex situ nanoindentation, ~1 GPa (considering a Tabor factor of 2.7 (ref. 40 ). The schematic in Fig. 4e illustrates the observed dislocation may reside initially on either a or plane, before gliding and depositing the loop observed in Fig. 4d . In twinned Al, the ITB migration-accommodated plasticity at greater stress can be explained by the interface disconnection glide mechanism revealed by MD simulations [14] . First, lattice dislocations dissociate at the ITB, causing its migration accompanied by load drop. Next, an interface disconnection dipole or loop nucleated at the ITB under high shear stress (parallel to the ITB), and the growth of interface disconnections can lead to ITB migration. Short steps or kinks consisting of ITB/CTB junctions are less stable energetically than straight ITBs [41] , and are likely sites for easier migration. The ITB segment in nt Al showed an instantaneous migration velocity of ~8 nm s −1 from our in situ studies. The high stress (500 MPa) at which ITB migrates implies that nt Al should have high strength as well as ITB accommodated plasticity. In summary, in situ nanoindentation study coupled with MD simulations reveal that ITBs in nt Al can effectively resist the pile-up of dislocations, and lead to significant work hardening. Repetitive dislocation-ITB interactions induce steps, where dislocation transmission eventually occurs, and ITB steps migrate to further accommodate plasticity at high stresses. This study provides a significant step forward toward a quantitative understanding of ITB-dominated plasticity in high strength, high SFE twinned metals, which could have wide spread applications. Sample preparation and in situ nanoindentation experiments We fabricated nt Al films by using a template technique [26] , [27] . To summarize, Al was deposited by magnetron sputtering onto an epitaxial nt Ag seed layer, and twins in Ag were replicated across the Ag/Al interface into Al via epitaxial growth. Cross-section TEM specimens were prepared by mechanical grinding and polishing, followed by low-energy ion milling. Samples were examined in a JEOL JEM-2010 TEM operated at 200 kV. A Nanofactory in situ nanoindentation holder with a spherical nanoindenter tip (measured radius ~200 nm) was used to examine deformability of nt Al. Indentation stress was estimated using the Hertzian contact estimation for the spherical tip [42] . A piezoelectric actuator controlled the specimen position in three dimensions. During indentation the indenter was fixed, and the specimen was advanced at a rate of 1 nm s −1 . Force–displacement information and movies were recorded during indentation, and still TEM micrographs were collected between tests. Estimated measurement error in force and displacement was ±5%. The calculation method for indentation stress has been presented in several of our recent in situ nanoindentation studies [39] , [43] . The following is a brief recap of the methodology used in this study. Estimation of projected area, a , based on spherical tip geometry (Hertzian contact, used in this manuscript): where R is the tip radius, D is indentation depth, t is foil thickness, F is indentation load and σ is indentation stress. In this manuscript, t is measured to be 30 nm. R is 200 nm, thus indentation stress can be calculated with known force and indentation depth. MD simulations MD simulations were conducted to study the details of dislocation-ITB interactions. For indentation testing in Al and Cu, we adopted the periodic boundaries for both the x and z axes. All ITB planes are the x – y planes. Each column has dimensions of 16 nm along the x axis, 60 nm along the y axis and 3 nm along the z axis. The radius of the indenter is 7.0 nm. MD simulations were conducted at temperature of 50 K with indentation velocity of 5 m s −1 . To explore the migration and step formation mechanisms, we also performed MD simulations in an Al bicrystal model ( Supplementary Fig. 4 ) at a temperature of 50 K. For the Al bicrystal simulation, the grain boundary plane is the x – y plane. The periodic boundary condition was adopted for the z axis, and all dislocations have the line sense parallel to the z axis. The flexible boundary conditions were used for both the x and y axis to mimic the study in an infinite bicrystal. The two dimensions for both grains are Lx =16 nm and Ly =64 nm, respectively. The thickness along the z axis, Lz , is 3 nm. Three dislocations were introduced in the right grain. All dislocations have Burgers vector of . During MD simulations, the bicrystal was subjected to a shear stress of 200 MPa parallel to the ITB plane. How to cite this article : Bufford, D. et al. In situ nanoindentation study on plasticity and work hardening in aluminium with incoherent twin boundaries. Nat. Commun. 5:4864 doi: 10.1038/ncomms5864 (2014).